Emergence of bimodality in controlling complex networks Our ability to control complex systems is a fundamental challenge of contemporary science. Recently introduced tools to identify the driver nodes, nodes through which we can achieve full control, predict the existence of multiple control configurations, prompting us to classify each node in a network based on their role in control. Accordingly a node is critical, intermittent or redundant if it acts as a driver node in all, some or none of the control configurations. Here we develop an analytical framework to identify the category of each node, leading to the discovery of two distinct control modes in complex systems: centralized versus distributed control. We predict the control mode for an arbitrary network and show that one can alter it through small structural perturbations. The uncovered bimodality has implications from network security to organizational research and offers new insights into the dynamics and control of complex systems. A dynamical system is controllable if it can be driven from any initial state to any desired final state within finite time [1] , [2] , [3] , [4] . In general, controllability can be achieved by changing the state of a small set of driver nodes, which drive the dynamics of the whole network [5] . For a linear time-invariant dynamics we can identify the minimum driver node set (MDS), representing the smallest set of nodes through which we can yield control over the whole system [5] , [6] , [7] , [8] , [9] , [10] , [11] , [12] , [13] , [14] , [15] , [16] , [17] , [18] , [19] . Although the number of driver nodes sufficient and necessary for control ( N D ) is primarily fixed by the network’s degree distribution, there are multiple MDSs with the same N D that can maintain control. For example, for the five node network shown in Fig. 1a N D =3, but the formalism indicates that control can be achieved via three different MDSs: {1,3,4}, {1,3,5} and {1,4,5}. 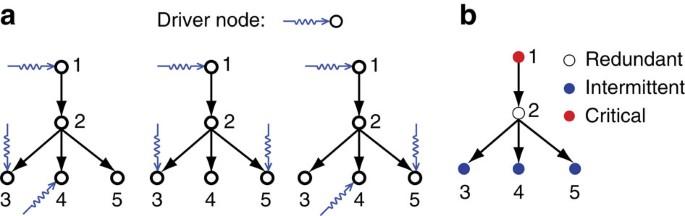Figure 1: Categories of driver nodes in a complex network. (a) A network with five nodes that can be control via three driver nodes (ND=3). The system is characterized by three distinct MDSs. (b) Node 1 is critical as it is part of all MDSs shown ina, node 2 is redundant as it does not participate in any MDS and nodes 3, 4, 5 are intermittent, participating in some but not all MDSs. Figure 1: Categories of driver nodes in a complex network. ( a ) A network with five nodes that can be control via three driver nodes ( N D =3). The system is characterized by three distinct MDSs. ( b ) Node 1 is critical as it is part of all MDSs shown in a , node 2 is redundant as it does not participate in any MDS and nodes 3, 4, 5 are intermittent, participating in some but not all MDSs. Full size image Here we explore the role of individual nodes in controlling a network by classifying each node into one of the three categories based on its likelihood of being included in MDS [20] : critical, meaning that a node must always be controlled to control a system (it is part of all MDSs); redundant, meaning that it is never required for control (does not participate in any MDSs) and intermittent, meaning that it acts as driver node in some control configurations, but not in others. For example, in Fig. 1a node 1 is critical, node 2 is redundant and nodes 3, 4, 5 are intermittent ( Fig. 1b ). This classification leads to the discovery of a bifurcation phenomenon, predicting that a bimodal behaviour determines the controllability of many real networks. This bimodality helps us uncover two control modes, centralized versus distributed. We demonstrate both analytically and numerically the existence of these two modes and show that the predicted control modes naturally emerge in a wide range of real networks. Identifying node categories We developed an algorithm to identify the redundant nodes in a network with N nodes and L links in steps, offering the fraction n r of redundant nodes for an arbitrary network (see Methods). We also proved that a node is critical if and only if it has no incoming links ( Supplementary Note 1 ), a theorem that provides the fraction of critical nodes in a network as n c = P in (0), where P in ( k ) is the incoming degree distribution. Finally, intermittent nodes are neither critical nor redundant, hence their fraction is n i =1− n c − n r . Bimodality in control To explore the role of the network topology, we measured n r and n c for networks with varying average degree ‹ k ›. We find that for small ‹ k › for an ensemble of networks with identical degree distribution P ( k ), n r and n c follow narrow distributions ( Fig. 2a ). This means that n r and n c are primarily determined by P ( k ) (refs 21 , 22 , 23 , 24 ). Surprisingly, when ‹ k › exceeds a critical value k c (ref. 25 ), P ( n r ) becomes bimodal, implying that systems with the same P ( k ) can exist in two distinct states: some have small n r and for others n r is very large. This bimodality is present in both random [26] and scale-free networks [27] , [28] ( Supplementary Note 2 ). The emergence of this bimodal behaviour is best captured by plotting n r versus ‹ k ›, observing a bifurcation as ‹ k › reaches k c ( Fig. 2b ). 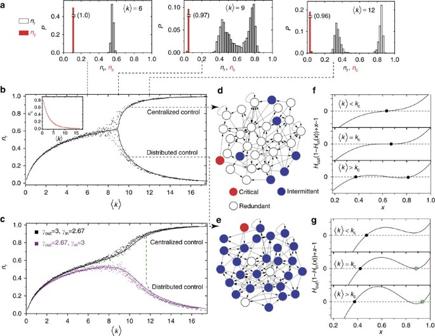Figure 2: Bifurcation in control. (a) Distribution of the fraction of redundant (nr) and critical (nc) nodes in scale-free networks withγout=γin=3, documenting the emergence of a bimodal behaviour for high ‹k›. (b)nrandnc(insert) versus ‹k› in scale-free networks with degree exponentsγout=γin=3, illustrating the emergence of a bifurcation for high ‹k›. (c)nrin scale-free networks with asymmetric in- and out-degree distribution, that is,γout=3,γin=2.67 (upper branch) andγout=2.67,γin=3 (lower branch). The control mode is predetermined by their degree asymmetry. The solid lines inbandccorrespond to the analytical prediction of equations (1) and (2). The dashed line is the discontinuous solution of equation (2) whenγout=3 andγin=2.67, which shows a gap between the actual evolution ofnr. (d,e) Networks displaying centralized and distributed control. For both networksND=4 andNc=1, yet they have rather different number of redundant nodes,Nr=23 indandNr=3 ine. (f,g) The curvesHout(1−Hin(x))+x−1 from equation (2) shown for different ‹k›,γout=γin=3 infandγout=3,γin=2.67 ing. The continuous stable solutions of equation (2) are shown as filled dots and the discontinuous solutions as empty circles. This bifurcation predicts two distinct control modes: Figure 2: Bifurcation in control. ( a ) Distribution of the fraction of redundant ( n r ) and critical ( n c ) nodes in scale-free networks with γ out = γ in =3, documenting the emergence of a bimodal behaviour for high ‹ k ›. ( b ) n r and n c (insert) versus ‹ k › in scale-free networks with degree exponents γ out = γ in =3, illustrating the emergence of a bifurcation for high ‹ k ›. ( c ) n r in scale-free networks with asymmetric in- and out-degree distribution, that is, γ out =3, γ in =2.67 (upper branch) and γ out =2.67, γ in =3 (lower branch). The control mode is predetermined by their degree asymmetry. The solid lines in b and c correspond to the analytical prediction of equations (1) and (2). The dashed line is the discontinuous solution of equation (2) when γ out =3 and γ in =2.67, which shows a gap between the actual evolution of n r . ( d , e ) Networks displaying centralized and distributed control. For both networks N D =4 and N c =1, yet they have rather different number of redundant nodes, N r =23 in d and N r =3 in e . ( f , g ) The curves H out (1− H in ( x ))+ x −1 from equation (2) shown for different ‹ k ›, γ out = γ in =3 in f and γ out =3, γ in =2.67 in g . The continuous stable solutions of equation (2) are shown as filled dots and the discontinuous solutions as empty circles. Full size image Centralized control: for networks that follow the upper branch of the bifurcation diagram most nodes are redundant ( n r ). This means that in these networks one can achieve control through a small fraction of all nodes ( n c + n i ), hence capturing a centralized control mode ( Fig. 2d ). This has obvious consequences in communication systems, as one can ensure a centralized system’s security by protecting only a small fraction of nodes ( n c + n i ); in an organizational setting centralized network may be better suited for task execution, such as manufacturing, where efficiency is enhanced by subordination to a small number of control nodes. Distributed control: for networks on the lower branch n c + n i can exceed 90% of the nodes. Hence, most nodes can act as driver nodes in some MDSs, resulting in a distributed control mode ( Fig. 2e ). Securing such distributed communication networks requires significant resources, as one can gain control of the system via a large number of control configurations. Yet organizations displaying distributed control may be more capable of harbouring innovation, as different node combinations could take control of the organization’s direction. Intuitively, one would expect these two different control modes to be associated with distinct network properties. However, we find that networks with identical in- and out-degree distribution can develop centralized or distributed control modes with equal probability ( Fig. 2a ). For networks with different in- and out-degree distributions the symmetry between the two branches is broken, forcing the network in one or the other branch of the bifurcation diagram. This is illustrated for networks with and , where γ in ≠ γ out . The degree asymmetry forces a network to follow one or the other branch of the bifurcation diagram ( Fig. 2c ), predetermining whether the network displays a centralized or a distributed control mode. Analytical approach To understand the origin of the observed control modes, we map the control problem to maximum matching [5] , [29] (see Methods), which provides the fraction of redundant nodes in infinite networks as where is the generating function for P in ( k ) (ref. 22 ). Here θ out is the solution of the recursive equation where and Q out,in ( k )= P out,in ( k ) × k /‹ k › is the excess degree distribution. Equations (1) and (2) self-consistently predict n r from the network’s degree distribution, in excellent agreement with the numerical results (see the continuous lines in Fig. 2b ), helping us understand the origin of the observed bifurcation. For P in ( k )= P out ( k ) equation (2) has a single solution for small ‹ k › (top panel in Fig. 2f ). As ‹ k › reaches k c , equation (2) develops three solutions, two of which are stable, corresponding to the two branches of the bifurcation diagram. As the new solutions are an analytic continuation of the ‹ k ›< k c solution, the system can continue in any of the two branches, hence, the centralized or the distributed control modes are equiprobable. If, however, P in ( k )≠ P out ( k ), for ‹ k ›> k c only one of the two stable solutions is an analytical continuation of the prebifurcation solution (middle panel in Fig. 2g ). In other words infinite systems with different P out ( k ) and P in ( k ) are destined for the centralized or distributed control mode, corresponding to the two branches of the bifurcation diagram, depending on the nature of their degree asymmetry. For small systems, the two modes can coexist and jumps between them are possible ( Supplementary Figs S1 and S2 ). Bimodality in real networks To demonstrate the empirical relevance of these tools, we used equations (1) and (2) to calculate n r for several real networks, starting from their degree distribution ( Supplementary Tables S1 and S2 ). Note that while for some of these networks control is of potential relevance (like regulatory networks [30] , [31] , [32] or neural networks [33] ), others like citation networks [34] , [35] , [36] or the WWW [37] , [38] , [39] are of little or no relevance for control. We analyse them mainly because they offer diverse topologies that test the limits of our predictions. We obtain a reasonable agreement between the analytically predicted and N r obtained directly for each network ( Fig. 3a , Supplementary Fig. S3 ). To compare n r for different networks, we plot them in function of 1− n D , representing the fraction of nodes that do not require external control. Obviously, real networks have widely different degree distributions, degree asymmetries and even potential correlations [40] , [41] , [42] , [43] , [44] , [18] . Despite these the predicted bifurcation is observed in real systems as well ( Fig. 3b , Supplementary Fig. S4 ). We find that some network structures, such as the E. coli metabolic network [45] , are in the ‘prebifurcation’ region ‹ k ›< k c : others, such as the mobile call network [46] , [47] , [48] , [49] , [50] and citation networks [34] , [35] , [36] , follow one or the other branch of the bifurcation diagram, indicating that they are characterized by either centralized or distributed control. To identify the control mode charactering a particular network, we introduce the transpose network, whose wiring diagram is identical to the original network but the direction of each link is reversed. The control mode is captured by comparing n r of a network with of its transpose network: if a network is centralized and if Δ n r <0 it is distributed ( Supplementary Note 3 ). We find that a network’s degree distribution allows us to infer its control mode ( Supplementary Note 4 ). 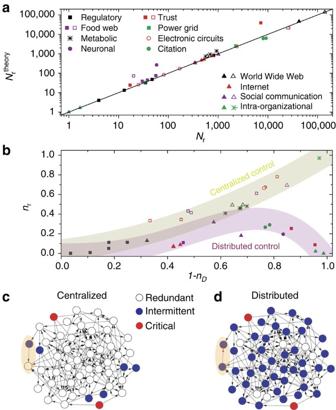Figure 3: Bimodality in real networks. (a) The number of redundant nodesNrin real networks (Supplementary Tables S1 and S2) and the theoretical prediction of equations (1) and (2). Hollow symbols represent networks characterized by centralized control (Δnr>0) and solid symbols correspond to the distributed control mode (Δnr<0). For networks marked with a star symbol, Δnr≈0 and the control mode can not be identified. (b)nrversus 1−nDfor real networks. The networks follow the two branches corresponding to centralized and distributed control (highlighted bands). (c) A network in the centralized control mode. (d) After flipping the direction of one link inc(highlighted in bothcandd), the control configuration changes from centralized to distributed mode. For both networksND=5 andNc=2, but in the centralized mode 8 nodes have a role in control (2 critical plus 6 intermittent) while in the distributed mode 43 nodes are engaged in control (2 critical plus 41 intermittent). Figure 3: Bimodality in real networks. ( a ) The number of redundant nodes N r in real networks ( Supplementary Tables S1 and S2 ) and the theoretical prediction of equations (1) and (2). Hollow symbols represent networks characterized by centralized control (Δ n r >0) and solid symbols correspond to the distributed control mode (Δ n r <0). For networks marked with a star symbol, Δ n r ≈0 and the control mode can not be identified. ( b ) n r versus 1− n D for real networks. The networks follow the two branches corresponding to centralized and distributed control (highlighted bands). ( c ) A network in the centralized control mode. ( d ) After flipping the direction of one link in c (highlighted in both c and d ), the control configuration changes from centralized to distributed mode. For both networks N D =5 and N c =2, but in the centralized mode 8 nodes have a role in control (2 critical plus 6 intermittent) while in the distributed mode 43 nodes are engaged in control (2 critical plus 41 intermittent). Full size image Altering the control mode The fact that the two control modes are better suited for different tasks raises an important question: can we turn a network initially in the centralized mode into a network in the distributed mode, or the other way around? Such a transition is achieved by the transpose network. Indeed, we can show that if the original network has a distributed control mode, its transpose will be centralized. Yet, in most real systems switching the direction of all links is either impossible or infeasible. We find, however, that in some networks the transition can be induced by local changes, in some cases requiring us to flip the direction of only a single well-chosen link ( Fig. 3c ). The precise local change required to induce the transition is determined by the network’s size and degree asymmetry: the larger the network or the higher degree asymmetry, the more links need to be altered to induce this transition. For example, for two manufacturing and consulting networks [51] ( N =77, L =2228 and N =46, L =858) the control mode can be altered by flipping only one link. In contrast for the prison inmate network [52] , [53] , food web in Little Rock lake [54] and the C. elegans neural network [33] , we need to change the direction of several links (4, 17 and 54 respectively, representing 2%, 0.7% and 2% of all links) to alter the control mode. In summary, our attempts to quantify the role of individual nodes have led us to an unexpected discovery: the existence of two distinct control modes, whose emergence is governed by a bifurcation phenomenon. The control mode is determined by the system’s degree asymmetry and has immediate implications on network security or efficiency in organizational settings. Most importantly, bimodality is a general property of all dense networks, hence, we must consider its implications each time we wish to control a complex system with sufficient connectivity. These results raise several intriguing questions. For example, the finding that the control mode can be altered via structural perturbations raises the need for tools to identify the minimum number of links whose reversal can help us reach the desired control mode [55] . Furthermore, the proposed node classification raises the possibility to correlate the role of a node in control with the intrinsic node attributes. Finally, our node classification is based on the node’s participation in various MDSs. However, one can explore other node classifications as well, like that based on the energy needed for control, or the time necessary to reach the final state [9] , important issues that need further investigation. Although bimodality is ubiquitous in physics, chemistry and biology, the finding that it also has a key role in network control opens new avenues to explore the control of real systems. Identifying the driver nodes We convert a directed network into a bipartite graph with two disjoint sets of out and in nodes. A directed link from node i to j corresponds to a connection between node i in the out set and node j ' in the in set ( Supplementary Fig. S5 ). By finding the maximum matching of the bipartite graph, the minimum driver nodes are unmatched nodes in the in set. The critical, intermittent and redundant nodes are always matched, occasionally matched and never matched nodes in the in set, respectively ( Supplementary Note 5 ). Identifying the redundant nodes Redundant nodes are always matched in the bipartite graph. Therefore, if we force them unmatched, there would be no alternative matching and the number of matched nodes will decrease, inspiring the algorithm we developed to identify them: (1) Find the maximum matching of the bipartite graph using the Hopcroft–Karp algorithm [29] , [56] , [57] , [58] , [59] . Obtain a set of matched nodes in the in set (denoted by M ). (2) Pick one element (denoted by node i ) in M . Identify the node in the out set that matches node i (denoted by node j ). (3) Keep the current matching and temporarily remove node i with all its links. Check if there is an augmenting path [58] , [29] that starts from node j , ends at an unmatched node and alternates between unmatched and matched links on the path. (4) If no augmenting path is found, node i needs to be always matched, therefore, it is redundant. Otherwise node i is replaceable and hence it is intermittent. (5) Add back the removed node i and repeat step 2 until all nodes in set M is tested. The number of computational steps needed to find one maximum matching is . Each matched node requires a breadth first search ( time) for the augmenting path. The number of matched nodes is proportional to N . Therefore, the complexity of this algorithm is . Calculating n r analytically Denote with G a bipartite graph and G ′= G \ i the subgraph of G obtained by removing node i and all its links ( Supplementary Fig. S6 ). We proved a theorem that node i is not always matched in G if and only if all its neighbouring nodes are always matched in the subgraph G ′ ( Supplementary Note 6 ). On the basis of this theorem, the probability that a node in the in set with degree k is not always matched is p k ,in =( θ out ) k where θ out is the probability that a neighbouring node is always matched in the out set of the subgraph G ′. When averaging over degree distributions in infinite networks, the fraction of redundant nodes, which are always matched nodes in the in set, is which gives equation (1). In the construction of subgraph G ', a neighbour of node i is accessed through a randomly chosen link. This implies that the degree distribution associated with the neighbouring node is the excess degree distribution, that is, the degree distribution for a node at the end of a randomly chosen link. Furthermore, in G ′ this randomly chosen link is excluded, meaning that the degree of the neighbouring nodes will be less by 1. Therefore, θ out satisfies the equation By substituting in for out, we can build a similar equation Combining equations (4) and (5), we obtain equation (2). Networks analysed The model networks in this paper are Erdös–Rényi network [26] and scale-free network [27] , [28] , generated via the static model [60] . The real networks we explored are described in Supplementary Tables S1 and S2 . How to cite this article: Jia, T. et al. Emergence of bimodality in controlling complex networks. Nat. Commun. 4:2002 doi: 10.1038/ncomms3002 (2013).